Inner gorges cut by subglacial meltwater during Fennoscandian ice sheet decay The century-long debate over the origins of inner gorges that were repeatedly covered by Quaternary glaciers hinges upon whether the gorges are fluvial forms eroded by subaerial rivers, or subglacial forms cut beneath ice. Here we apply cosmogenic nuclide exposure dating to seven inner gorges along ~500 km of the former Fennoscandian ice sheet margin in combination with a new deglaciation map. We show that the timing of exposure matches the advent of ice-free conditions, strongly suggesting that gorges were cut by channelized subglacial meltwater while simultaneously being shielded from cosmic rays by overlying ice. Given the exceptional hydraulic efficiency required for meltwater channels to erode bedrock and evacuate debris, we deduce that inner gorges are the product of ice sheets undergoing intense surface melting. The lack of postglacial river erosion in our seven gorges implicates subglacial meltwater as a key driver of valley deepening on the Baltic Shield over multiple glacial cycles. Rivers at the margins of decaying ice masses carry water and sediment in prodigious amounts that vary with seasonal fluctuations in melt rate and the hydraulic efficiency of supra and subglacial drainage systems [1] , [2] , [3] . Such rivers frequently occupy V-shaped inner bedrock gorges whose origin has fuelled a long-standing debate with links to a broader discussion on the erosional efficacy of rivers versus glaciers [4] , [5] , [6] , [7] . Fluvial sediment loads measured at the ice front provide the pivotal evidence for significant subglacial erosion [6] , [7] , but how much of this erosion is the work of ice, and how much the work of subglacial meltwater? Moreover, most acknowledge that it is generally uncertain whether sediment yield reflects contemporary erosion of bedrock, or remobilisation of debris generated long ago under different boundary conditions [2] , [7] . Erosion patterns under continental ice sheets reflect basal thermal regimes [4] , [8] , [9] , [10] . Minimal erosion across interfluves and uplands where ice is commonly frozen to the bed contrasts with areal scouring or selective linear erosion along valleys where ice thickens and accelerates [9] , [11] , [12] , [13] , [14] . Preservation of pre (last) glacial surfaces is no longer controversial thanks to in situ cosmogenic nuclide measurements that indicate long-term nuclide accumulation over extensive areas of non-glacial blockfields [10] , [11] , [12] , [13] , [14] . In the valleys, however, understanding the partitioning and timing of glacial and fluvial erosion has proved more challenging because morphological and cosmogenic nuclide-based evidence for glacial or fluvial activity is strongly overprinted or erased during successive glacial cycles [12] . Inner gorges display ‘valley-in-valley’ cross-sections and frequently host a mixture of subglacial and subaerial bedforms that suggest a dynamic intersection of glacial and fluvial regimes [15] , [16] , [17] , [18] , [19] , [20] . Explanations for inner gorge formation divide into those favouring subglacial processes versus those that invoke subaerial rivers operating either in postglacial or preglacial (interglacial) times. The notion of channelized subglacial meltwater acting as the primary erosional agent is rooted in early Scandinavian studies [15] , [21] , [22] , and continues to receive strong support among those concerned with tunnel valley genesis [23] , [24] . Typical field evidence for subglacial meltwater erosion includes anastomosing channels, irregular valley long profiles and topography that amplifies hydraulic potential [2] , [9] , [18] , [20] . Secondly, other workers attribute inner gorges to subaerial pre or postglacial river incision in response to base-level fall or shifts in sediment supply [25] , [26] , [27] , [28] . A third explanation sees inner gorges as palimpsest fluvial forms whose relief can deepen over multiple glacial cycles. As reported from sites in the European Alps, preglacial inner gorges might become plugged with debris during glacial advances followed by flushing by subaerial rivers that carve incrementally deeper into bedrock [19] , [29] , [30] . Our study adopts a fresh approach for understanding fluvial erosion associated with glaciation by applying in situ cosmogenic nuclide exposure dating to inner gorges on a large spatial scale. We examine gorges developed along ~500 km of the former Fennoscandian ice sheet margin in northern Sweden ( Figs 1 and 2 ). We aim to test whether the inner gorges represent predominantly inherited forms, or were carved subglacially, and whether the rivers have been actively eroding in the Holocene. Inner gorges with preglacial origins would be expected to yield exposure ages predating deglaciation (>10 kyr, Fig. 1a ), whereas those formed or deepened subglacially would yield exposure ages tied to the advent of ice-free conditions. Postglacial river erosion would be indicated by gorge surfaces becoming younger with depth. 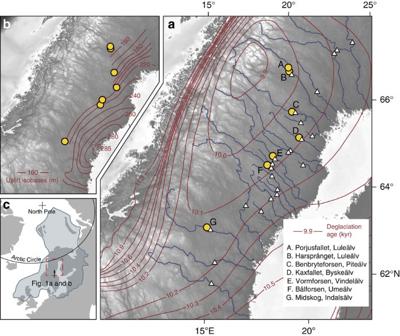Figure 1: Field area in northern Scandinavia. (a) 24 study rivers (blue lines) and seven inner gorges (yellow dots labelled A to G) sampled for exposure dating. Glaciofluvial deltas (white triangles) associated with the highest and most inland shorelines mark where the ice margin and terrestrial coastline briefly coexisted before the ice retreated inland. Deglaciation isochrons (red) indicate the tempo of ice margin retreat (see Methods). (b) Isobases (red) indicate elevations of uplifted postglacial shorelines33relative to the sampled inner gorges (yellow dots) that span ~500 km of the palaeo-ice sheet margin. Note that individual isobases are time-transgressive because ice-free conditions necessary for shoreline development progressed from south to north; their concentric pattern reflects isostatic loading of the ice sheet, with maximum ice thickness close to the present-day coast. (c) Maximum extent of the Fennoscandian ice sheet at the Late Weichselian glacial maximum ~20 kyr (ref.54). Figure 1: Field area in northern Scandinavia. ( a ) 24 study rivers (blue lines) and seven inner gorges (yellow dots labelled A to G) sampled for exposure dating. Glaciofluvial deltas (white triangles) associated with the highest and most inland shorelines mark where the ice margin and terrestrial coastline briefly coexisted before the ice retreated inland. Deglaciation isochrons (red) indicate the tempo of ice margin retreat (see Methods). ( b ) Isobases (red) indicate elevations of uplifted postglacial shorelines [33] relative to the sampled inner gorges (yellow dots) that span ~500 km of the palaeo-ice sheet margin. Note that individual isobases are time-transgressive because ice-free conditions necessary for shoreline development progressed from south to north; their concentric pattern reflects isostatic loading of the ice sheet, with maximum ice thickness close to the present-day coast. ( c ) Maximum extent of the Fennoscandian ice sheet at the Late Weichselian glacial maximum ~20 kyr (ref. 54 ). Full size image The highest shorelines and glaciofluvial deltas The demise of the Fennoscandian ice sheet ( Fig. 1 ) was a time of major interplay between glacioisostasy and eustatic sea level rise [31] , [32] , [33] , [34] , [35] . This interplay directed the timing and position of the earliest coastal emergence and formation of the ‘highest shorelines’ (the marine limit) and glaciofluvial deltas in northern Sweden ( Fig. 1a ), which we use as important markers in the landscape (see Methods). Owing to spatial and temporal differences in glacioisostatic adjustments and sea level rise over successive glacial cycles, the marine limits are unlikely to be coincident for successive deglaciations [33] , [34] , [35] . Glaciofluvial deltas associated with the shorelines have been used widely to reconstruct spatial patterns of glacioisostatic rebound and to constrain maximum ice sheet thickness [31] , [32] , [33] , [34] , [35] ( Fig. 1b ). Rivers supplied debris to build glaciofluvial deltas ( Fig. 1a ), which rapidly migrated coastward in the wake of falling base level [33] , [34] , [35] owing to glacioisostatic uplift outpacing eustatic sea level rise. We mapped the inland limits of the highest shoreline and glaciofluvial deltas in 24 valleys along the palaeo-coast that marked the last ice sheet’s eastern margin ( Fig. 1a ). Inner gorges were commonly found downstream of glaciofluvial channels and close to deltas that mark the marine limit ( Fig. 1a ), suggesting a common timing in their development. Six well-developed inner gorges were selected along large mainstem rivers ( Supplementary Figs 1–14 and Supplementary Table 1 ), and bedrock surfaces were sampled for in situ cosmogenic 10 Be analysis. To test whether there was any direct relation between gorge formation and the marine limit, we also sampled a gorge at Porjusfallet (Luleälv), 10 km inland from the marine limit. 10 Be exposure ages Twelve of the fifteen 10 Be exposure ages are generally consistent with the timing of ice margin retreat ( Figs 1a and 3 ), strongly suggesting that bedrock erosion during the last glaciation removed the full 10 Be inventory. Three outlying exposure ages from surfaces marginal to the inner gorges (B1, K1, U1, Fig. 2 ) predate deglaciation by ~5.4–10.3 kyr, indicating that some fraction of their 10 Be inventory is inherited from a previous exposure period. The depth of erosion apparently varied over short distances, as seen at Benbryteforsen and Balforsen where sites with inherited 10 Be occur within 100 m of those reset by subglacial erosion ( Fig. 2c,f ). Details of the 10 Be sampling and analyses are reported in the Methods and Supplementary Tables 2–4 . 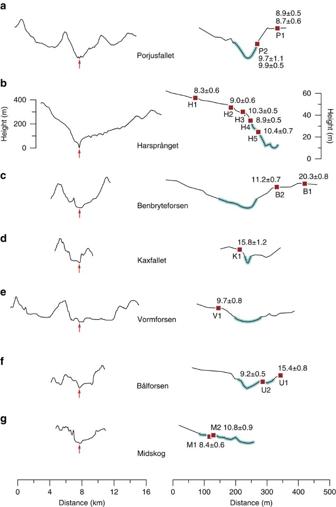Figure 2:10Be exposure ages and cross-sections. (a–g), Channel cross-sections (on right) are located by red arrows in the broader valley cross-sections (on left). Vertical scales apply column-wise and vertical exaggeration is 3.5 and 15 times on the right and left, respectively. All exposure ages (red squares) are given in kyr ±1σ internal uncertainty (note duplicates at Porjusfallet). The zone of active bedrock channel erosion (thick blue lines) pertains to the pre-dam flood regime, as estimated from stage indicators and the presence of lichen. Five samples were collected from the channel zone (P2, H5, U2, M1, M2), the latter two from the channel bed. Figure 2: 10 Be exposure ages and cross-sections. ( a – g ), Channel cross-sections (on right) are located by red arrows in the broader valley cross-sections (on left). Vertical scales apply column-wise and vertical exaggeration is 3.5 and 15 times on the right and left, respectively. All exposure ages (red squares) are given in kyr ±1σ internal uncertainty (note duplicates at Porjusfallet). The zone of active bedrock channel erosion (thick blue lines) pertains to the pre-dam flood regime, as estimated from stage indicators and the presence of lichen. Five samples were collected from the channel zone (P2, H5, U2, M1, M2), the latter two from the channel bed. Full size image The regional concordance between exposure ages and deglaciation ( Fig. 3 ) along the ~500 km palaeo-coast is the strongest evidence for gorges being extensively modified before or during deglaciation. 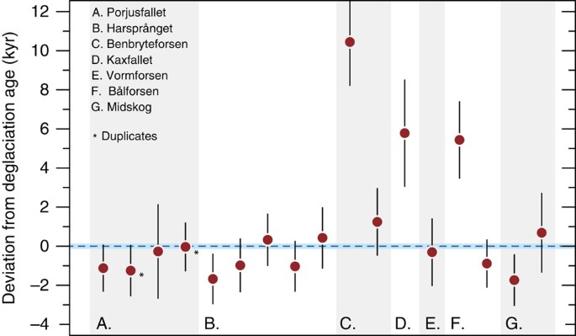Figure 3:10Be exposure ages expressed as deviations from deglaciation age. Negative deviation means that exposure ages are younger than deglaciation, and all ages are shown with ±2σ external uncertainty. Vertical bands separate the field sites. Isochron uncertainty (±150 y) is indicated by the blue band. Deviations calculated using an alternative isochron map36yield similar results (seeSupplementary Table 3, and Methods for full details of the deglaciation model). The match is equally good using an alternative deglaciation map [36] ( Supplementary Table 3 ). The margins of uncertainty associated with our deglaciation isochrons (±150 y, ~1%, see Methods) and exposure ages (~5–9% external uncertainty) means that we cannot exclude the possibility that some inner gorges were affected by catastrophic subaerial water flows generated by collapse of glacially-dammed lakes during deglaciation [18] , [37] ; however, there is no evidence of such events in the vicinity of the gorges we examined. On the other hand, because the ice sheet blocks cosmic radiation, subglacial erosion is entirely compatible with the lack of systematic relation between exposure age and height above the channel zone ( Fig. 2 ), and consistent with a model in which the gorges emerged fully formed at the retreating ice front. Postglacial fluvial erosion, which would yield ages younging towards the active channel zone, is likewise discounted; four of five channel zone samples (from four separate gorges, excluding sites with 10 Be inheritance located outside inner gorges at Benbryteforsen and Bålforsen, Fig. 2 .) yield exposure ages that correspond to deglaciation within 1σ external uncertainty. Nonetheless, given that just two measurements derive from the channel bed (M1 and M2, Fig. 2 ), we leave open the prospect of restricted postglacial erosion in keeping with previous views [31] , [38] . Figure 3: 10 Be exposure ages expressed as deviations from deglaciation age. Negative deviation means that exposure ages are younger than deglaciation, and all ages are shown with ±2σ external uncertainty. Vertical bands separate the field sites. Isochron uncertainty (±150 y) is indicated by the blue band. Deviations calculated using an alternative isochron map [36] yield similar results (see Supplementary Table 3 , and Methods for full details of the deglaciation model). Full size image We find no evidence to suggest that the inner gorges existed in their current form before the last Weichselian glacial advance, were filled with sediment during the advance and were then excavated subaerially [19] , [30] . No glacigenic sediments were found in the gorges, and any temporary cover (or stagnant ice) was too short-lived [8] to shield bedrock from cosmic rays enough to affect the exposure ages. The close agreement between the exposure ages and the timing of deglaciation ( Fig. 3 ) means that any such flushing of glacigenic valley-fill sediments debris must have occurred subglacially [2] , [19] , [30] . We cannot determine categorically what fraction of gorge depth (if any) was carved during a previous glacial or interglacial period. However, the lack of incision observed over the Holocene indicates that subaerial fluvial erosion is inefficient, and because shoreline positions are not likely to be reproduced in successive deglaciations, the correlation of gorges with the marine limit, if somehow causal, suggests that the gorges are deglaciation forms that were cut subglacially during decay of the last Fennoscandian ice sheet. From our focus on deglaciation events in northern Sweden we draw some pertinent links with the western margin of the Greenland ice sheet today where outlet glaciers also debouch onto a narrow terrestrial strip fringing the ablation zone. At Leverett Glacier (67.06°N, 50.17°W) satellite imaging of lake drainage events suggests that the seasonal increase in the hydraulic efficiency of subglacial drainage (that is, the capacity to erode the substrate via channelized flow) extends tens of kilometres inboard from the terminus, and surface meltwater is accessing the base of the ice sheet and evacuating debris at rapid rates [1] , [2] , [39] . In addition to the effects of subglacial hydrology on sliding velocity [2] , [40] , the expansion inboard of zones of subglacial erosion [1] is probably characteristic of decaying ice sheets [2] , [10] . 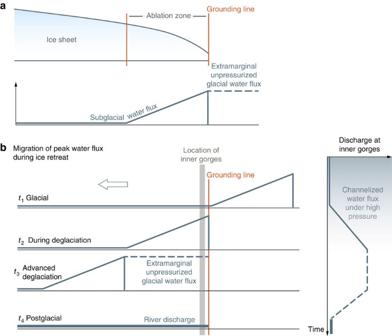Figure 4: Illustration of inner gorge formation relative to meltwater flux at the grounding line-margin of a decaying ice sheet. (a) Ice sheet margin in section showing the ablation zone and corresponding growth in subglacial meltwater flux. The inboard-migrating tip of the meltwater ‘wedge’ extends in the order of ~100 km inboard. (b) Inboard migration of the ablation zone drives a corresponding migration of peak meltwater flux across the landscape via surface melting of the ice sheet. The right panel is a notional illustration of the variation in meltwater flux through the gorges as deglaciation progresses from t1to t4. Subglacial meltwater flux at the gorge sites may be low when the ablation zone lies outboard of the gorge zone (t1), but rising as the ablation zone migrates across the gorge zone (t1–t2). Concurrently, high fluxes of channelized meltwater with elevated hydraulic potential gradient are forced along low-lying terrain corridors, flushing debris and promoting maximum bedrock erosion at t2. After further ice retreat (t3), high fluxes of meltwater continue until final deglaciation (t4), but in contrast to t2, erosion rates along the gorges decline because the subaerial rivers are unpressurized and sediment ‘tools’ necessary for bedrock erosion are largely trapped in proglacial lakes28. Figure 4 illustrates how inner gorges may be generated as a function of channelized meltwater flux at the margin of a retreating ice sheet. A point at the base of the Fennoscandian ice sheet ~100 km inboard from the margin would have been ice-free after ~100–170 y, assuming a retreat rate of 0.6–1.0 km y –1 ( Figs 1a and 4 ). Thus, development of subglacial inner gorges that are tens of metres deep implies extreme, though not implausible, erosion rates that we speculate signify intense meltwater activity [2] , [17] , [20] , [40] perhaps involving abrupt drainage of supraglacial lakes into the base of the ice sheet [24] , [39] . We strongly suspect that the transition in ice margin retreat from marine to terrestrial mode is somehow critical to the formation of gorges near the grounding line ( Fig. 4 ); however, a full understanding of the physics of ice sheet decay, especially regarding subglacial hydrology, is some way off [1] , [2] , [3] , [40] . What we can say with confidence is that the regional pattern of eskers in northern Sweden is evidence for an energetic and channelized subglacial meltwater system (see Supplementary Fig. 15 ). Given that eskers and rivers both run orthogonal to the retreating ice front, it seems that the bedrock topography underlying the ablation zone will inevitably steer channelized subglacial flow along low-lying corridors during rapid decay [2] , [18] , [40] ( Fig. 4 ). We see bedrock morphology and subglacial hydrology as being inherently coupled systems. Subglacial gorges may therefore be both a product and driver of a positive feedback for enhancing drainage efficiency wherever intense surface melting produces large volumes of meltwater. It is perhaps significant that within a few centuries of the inner gorges being cut, the Fennoscandian ice sheet had disappeared. Figure 4: Illustration of inner gorge formation relative to meltwater flux at the grounding line-margin of a decaying ice sheet. ( a ) Ice sheet margin in section showing the ablation zone and corresponding growth in subglacial meltwater flux. The inboard-migrating tip of the meltwater ‘wedge’ extends in the order of ~100 km inboard. ( b ) Inboard migration of the ablation zone drives a corresponding migration of peak meltwater flux across the landscape via surface melting of the ice sheet. The right panel is a notional illustration of the variation in meltwater flux through the gorges as deglaciation progresses from t 1 to t 4 . Subglacial meltwater flux at the gorge sites may be low when the ablation zone lies outboard of the gorge zone (t 1 ), but rising as the ablation zone migrates across the gorge zone (t 1 –t 2 ). Concurrently, high fluxes of channelized meltwater with elevated hydraulic potential gradient are forced along low-lying terrain corridors, flushing debris and promoting maximum bedrock erosion at t 2 . After further ice retreat (t 3 ), high fluxes of meltwater continue until final deglaciation (t 4 ), but in contrast to t 2 , erosion rates along the gorges decline because the subaerial rivers are unpressurized and sediment ‘tools’ necessary for bedrock erosion are largely trapped in proglacial lakes [28] . Full size image The lack of postglacial river erosion in our seven gorges leads us to the speculative proposal that subglacial meltwaters, not interglacial rivers, are a key driver of valley deepening on the Baltic Shield over multiple glacial cycles ( Fig. 5 ). But unlike alpine glacial settings, which tend to further entrench pre-Quaternary dendritic drainage patterns [19] , [20] , [30] , [41] , low-relief shield landscapes allow the locus of subglacial erosion to switch laterally between neighbouring valleys over successive glaciations ( Fig. 5 ). The resulting distribution of erosional work is compatible with the anabranching valley networks commonly observed in regions repeatedly covered by continental ice sheets [4] , [16] , [17] , [18] , [42] . 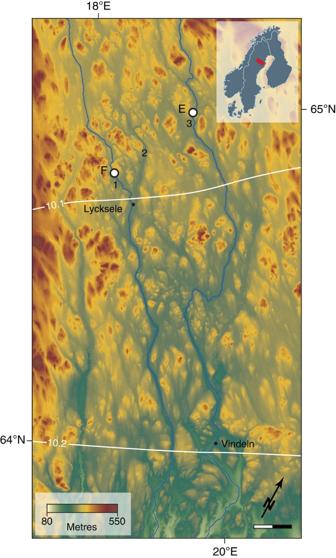Figure 5: Interconnected network of anabranching valleys in northern Sweden represented by a digital elevation model. Two rivers (blue lines) and inner gorge sites sampled for exposure dating: E, Vormforsen (Vindelälv); F, Bålforsen (Umeälv) (seeFig. 1a, and location inset); major glaciofluvial deltas are: 1, Betsele; 2, Dallundfältet; 3, Ruskträskfältet. Scale bar, 10 km. Deglaciation isochrons (white lines, kyr) indicate the alignment of the retreating ice margin relative to the anabranching valleys. Note the lack of tributary drainage; such interconnected valley networks are observed across much of the Baltic Shield42, suggesting that subglacial meltwater systems carve alternative lateral routes over multiple glaciations (Fig. 2e,fshows these valleys in cross-section; subglacial drainage paths are shown inSupplementary Fig. 15). Figure 5: Interconnected network of anabranching valleys in northern Sweden represented by a digital elevation model. Two rivers (blue lines) and inner gorge sites sampled for exposure dating: E, Vormforsen (Vindelälv); F, Bålforsen (Umeälv) (see Fig. 1a , and location inset); major glaciofluvial deltas are: 1, Betsele; 2, Dallundfältet; 3, Ruskträskfältet. Scale bar, 10 km. Deglaciation isochrons (white lines, kyr) indicate the alignment of the retreating ice margin relative to the anabranching valleys. Note the lack of tributary drainage; such interconnected valley networks are observed across much of the Baltic Shield [42] , suggesting that subglacial meltwater systems carve alternative lateral routes over multiple glaciations ( Fig. 2e,f shows these valleys in cross-section; subglacial drainage paths are shown in Supplementary Fig. 15 ). Full size image Deglaciation of the Fennoscandian ice sheet The isochron map describes the final ice retreat based on geomorphic mapping coupled with geochronology ( Fig. 1a,c ). Isochrons (±150 y uncertainty) are tied to the Swedish clay-varve chronology and correlated with the Greenland Ice Core Project (GRIP) chronology [43] , and the timing of final deglaciation is independently confirmed by cosmogenic exposure dating. The isochron map ( Fig. 1a , and Supplementary Fig. 16 ) was constructed as follows. Retreat-stage outlines are adjusted from Kleman [8] based on mapping by Hättestrand [44] of the youngest striae, till lineation directions and lateral meltwater channels ( Supplementary Fig. 15 )—following the rationale described in Kleman et al. [45] The geomorphology-based interpretation of the ice retreat pattern is linked to the Swedish clay-varve chronology at Pauträsk (locality shown in Supplementary Fig. 16 ; ref. 46 ). Connecting the clay-varve chronology to the present-day [47] yields 9,140 cal. yr BP for the ice margin at Pauträsk; to this we add 875 cal. yr according to the latest correlation of the clay-varve chronology with the GRIP chronology [43] , thereby giving a deglaciation age of 10,015 cal. yr BP at Pauträsk. For the timing of ice retreat from Pauträsk to the final ice remnants in the Kvikkjokk area (locality shown in Supplementary Fig. 16 ; ref. 8 ), we extrapolate the increase in retreat rate observed in the varve record, thereby yielding an estimated 9.9 kyr for the final deglaciation. As an independent check on the timing of final deglaciation, we compiled 26 cosmogenic exposure ages within 60 km of Kvikkjokk ( Supplementary Table 4 ), including boulder erratics ( n =22), bedrock surfaces from meltwater channels ( n =2), and lee-side scarps eroded during the last phases ( n =2) [13] , [48] , [49] , [50] , plus two unpublished ages). After rejecting seven samples with cosmogenic inheritance and one sample with incomplete exposure, the remaining 18 samples yielded a reduced χ 2 -value [51] of 1.48 for a weighted mean age of 10.2±0.7 kyr, an age that is within the uncertainty limits of the ~9.9 kyr obtained by extrapolating the clay-varve chronology. Additionally, we note that the concordance between exposure ages and deglaciation is equally good using the Boulton et al. [36] deglaciation chronology (comparative deviations are given in Supplementary Table 3 ). The inception of post-Younger Dryas (YD) ice retreat from southern Sweden is taken to match the timing of warming in Greenland at 11,525 cal. yr according to the GRIP chronology [43] , and carries an uncertainty of ±150 y (ref. 52 ). Our deglaciation isochron map is built upon the assumption that the floating Swedish clay-varve chronology [47] is internally correct for the region stretching from the YD limits (11,525 cal. yr) to Pauträsk (10,015 cal. yr). Hence, the Greenland ice core chronology is the chief source of isochron uncertainty (±150 y) from the YD limits to Pauträsk. For extrapolating the isochrons from Pauträsk to the final ice remnants at Kvikkjokk ( Supplementary Fig. 16 ), we aimed to fuse the chronological data with a retreat rate that is both glaciologically plausible and accordant with the field evidence. There is no a priori minimum rate of ice retreat (a static ice margin represents a ‘still-stand’); however, given neither end moraines nor evidence of large dead ice-masses [8] , nor cooling trends in the local biostratigraphy, we argue for a monotonic final decay. It is expected that the pace of ice margin retreat accelerated as final deglaciation was approached, because the accumulation area proportion of the ice sheet diminishes as the ice surface lowers. Yet, there are definite limits to the rate of melting, given realistic climatic conditions. Shifting the final deglaciation age to just 100 y older (that is, 10.0 kyr) requires an implausibly fast retreat rate from Pauträsk to Kvikkjokk of ~2 km y −1 , which represents a fourfold increase relative to the average ~0.5 km y –1 retreat rate from the YD limits to Pauträsk. A variation of 100 y falls within the ±150 y uncertainty associated with the isochrons linked to the varve chronology; hence, we maintain that ±150 y is a reasonable estimate of uncertainty on the deglaciation isochron map. We cannot exclude other sources of uncertainty related to identifying geomorphic evidence of deglaciation, but we consider such effects as probably small. Identification of the highest shorelines Guided by published sources [31] , [33] , [35] , we identified the inland limits of the highest elevation shoreline in each valley based on: (1) highest traces of wave erosion indicated by slopes washed bare of till; (2) downstream limits of ice-marginal glaciofluvial channels; and (3) highest glaciofluvial delta topsets. In 24 valleys ranging from ~150–350 m deep, inner gorges ~20 to 35 m deep ( Fig. 2 ) extend upstream of the inland limits of the highest shorelines ( Fig. 1a ). Valley cross-sections were constructed from a 50 m digital elevation model (Lantmäteriet); channel cross-sections were measured in the field with differential-GPS and assisted in most cases by rivers being impounded behind hydro-electric dams immediately upstream. Channel long profiles were derived from pre-dam surveys [53] (see Supplementary Fig. 1 ). 10 Be sampling and analyses From seven well-developed inner gorges cut in uniform granitic rocks, 15 smoothly abraded bedrock surfaces were sampled for 10 Be analysis. All samples were collected from flat to gently-inclined surfaces away from steep slopes, and above the highest shoreline so were never subject to significant water shielding. Five samples derive from the active channel zone (P2, H5, U2, M1, M2), the latter two from the channel bed. Quartz was isolated following standard procedures: 10 Be was extracted using ion chromatography at GFZ-Potsdam and the Glasgow University Cosmogenic Isotope Laboratory; 10 Be/ 9 Be ratios were measured at ETH-Zürich and SUERC AMS laboratories, including two sets of duplicates (that is, two separate aliquots measured from the same sample). See Supplementary Tables 2–4 for full details of the 10 Be analyses. How to cite this article: Jansen, J. D. et al. Inner gorges cut by subglacial meltwater during Fennoscandian ice sheet decay. Nat. Commun. 5:3815 doi: 10.1038/ncomms4815 (2014).